Biocompatibility of a genetically encoded calcium indicator in a transgenic mouse model Engineering efforts of genetically encoded calcium indicators predominantly focused on enhancing fluorescence changes, but how indicator expression affects the physiology of host organisms is often overlooked. Here, we demonstrate biocompatibility and widespread functional expression of the genetically encoded calcium indicator TN-XXL in a transgenic mouse model. To validate the model and characterize potential effects of indicator expression we assessed both indicator function and a variety of host parameters, such as anatomy, physiology, behaviour and gene expression profiles in these mice. We also demonstrate the usefulness of primary cells and organ explants prepared from these mice for imaging applications. Although we find mild signatures of indicator expression that may be further reduced in future sensor generations, the 'green' indicator mice generated provide a well-characterized resource of primary cells and tissues for in vitro and in vivo calcium imaging applications. Understanding calcium signals and their spatiotemporal regulation in complex tissues and organs is crucial for research on basic cell and organ function, disease states and for the development of pharmaceutical compounds [1] . Calcium imaging with fluorescent indicators has become a powerful tool for physiological studies in primary cells and tissues with high spatial and temporal precision [2] , [3] , [4] , [5] , [6] , [7] . Recently genetically encoded calcium indicators (GECIs) based on fluorescent proteins (FPs) have become valuable tools in studying calcium signalling in previously often intractable organelles, tissues and organisms [8] , [9] , [10] . Chronic long-term functional imaging studies with GECIs offer exciting new possibilities to follow physiological processes of cells and tissues as they differentiate, adapt to stimuli and degenerate due to ageing and disease. The engineering of GECIs has followed two major trends: the development of single fluorophore sensors that modulate fluorescence intensity of a single FP through calcium binding or that of indicators based on Förster resonance energy transfer (FRET). Latest generation sensors include the single fluorophore sensors G-CaMP3 and HS-G-CaMP [11] , [12] , [13] , and the FRET sensors YC 3.6, D3cpV and TN-XXL [14] , [15] , [16] . Although most engineering efforts focused on signal strength and optimization of expression, the long-term effects of chronic GECI expression on the host organism have not been studied in detail. Evidence for occasional interference between sensor and host cells has been reported. The calmodulin-based FRET sensors YC3.6 (ref. 14 ) and YC3.12 (ref. 17 ) were essentially inactivated during transgenic expression. Transgenic constitutive expression of the single fluorophore sensor G-CaMP2 in the mouse heart induced cardiomegaly, a pathological enhancement of heart size [18] , [19] . Calmodulin is a ubiquitous signalling protein with multiple levels of regulation [20] . To minimize these problems skeletal Troponin C (TnC) was used to generate FRET biosensors [21] , [22] , [23] . TnC is a calcium-binding protein specialized in regulating contraction in muscle. In contrast to earlier conflicting results skeletal muscle TnC was found to be exclusively expressed by skeletal muscle [24] , [25] , [26] , with no detectable expression in either neonatal or adult brain and other non-muscle tissues that were investigated [25] . Thus, calcium sensors based on TnC appear more bio-orthogonal in most tissues apart from muscle compared with calmodulin-based sensors. TN-XXL is the currently latest generation TnC-based calcium biosensor in which the amino terminal lobe of chicken skeletal muscle TnC was removed and the carboxy terminal lobe doubled to generate a sensor with high FRET change [16] . To establish a calcium-imaging mouse model that would provide access to a large variety of cell types and tissues we generated transgenic mice with the CAG promoter driving constitutive expression of TN-XXL globally in a majority of cell types within the organism. We characterized expression of the sensor in these mice and used microarray expression profiling, anatomical analysis, behavioural testing and measurements of basic physiological parameters to assess potential consequences of biosensor expression on the host organism and to validate the model for future applications. We demonstrate long-term stability of sensor expression, present an analysis of possible side effects of indicator expression on the host organism and show indicator functionality in a variety of tissues and cell types. Widespread expression of TN-XXL in transgenic mice From a C57BL/6 background we generated transgenic mice expressing TN-XXL under control of the ubiquitously active hybrid CMV enhancer/chicken β-actin (CAG) promoter [27] . To enhance expression of the calcium biosensor we included the Woodchuck post-transcriptional regulatory element (WPRE) [28] downstream of TN-XXL ( Fig. 1a ). Out of six founders the line with highest expression of TN-XXL was selected as determined by fluorescence imaging of dissected organs. Mice from this line showed normal longevity, fertility, body and litter sizes compared with their non-transgenic siblings (not shown). Western blot analyses using anti-green fluorescent protein (GFP) antibodies revealed an expression of TN-XXL in the majority of tissues ( Fig. 1b ). A single band at 69 kDa was seen in all tissues analysed, demonstrating stable expression of the indicator. In addition, fluorescence images of homozygous, heterozygous and wild-type newborn pups, a series of images of isolated organs and frozen sections confirmed the wide spread expression in organs, such as brain, skeletal muscle, heart, kidney, pancreas or liver ( Figs 1c,d ; Supplementary Fig. S1 ). Organ size was in all cases comparable between wild-type and homozygous transgenic mice ( Fig. 1d ), with the exception of heart. 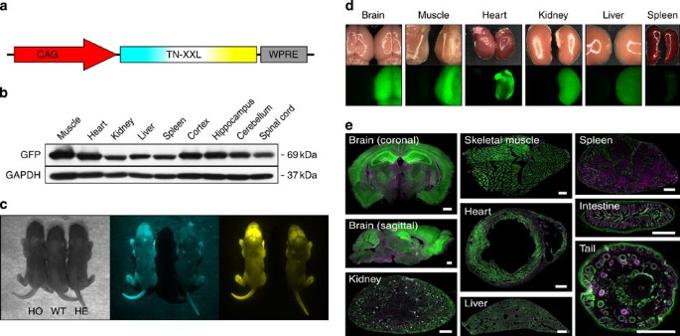Figure 1: Wide-spread expression of TN-XXL in tissues and organs of TN-XXL transgenic mice. (a) Scheme of the transgene construct with the CMV enhancer/chicken β-actin (CAG) promoter upstream, and the WPRE downstream of TN-XXL. (b) Western blot analysis of different tissue lysates using an anti-GFP antibody for the TN-XXL expression and an anti-GAPDH antibody as control. (c) Images of three newborn mice (HO, homozygous; HE, heterozygous; WT, wild-type) illuminated with bright field (monochrome), CFP (blue) and cpCitrine (yellow) fluorescence. (d) Bright field and fluorescence images of isolated organs from TN-XXL transgenic mice (right) compared with wild-type controls (left). (e) Overview of TN-XXL fluorescence (green) in frozen sections of several tissues co-stained with 4′,6-diamidino-2-phenylindole (DAPI; magenta) (Scale bars, 500 μm). Figure 1: Wide-spread expression of TN-XXL in tissues and organs of TN-XXL transgenic mice. ( a ) Scheme of the transgene construct with the CMV enhancer/chicken β-actin (CAG) promoter upstream, and the WPRE downstream of TN-XXL. ( b ) Western blot analysis of different tissue lysates using an anti-GFP antibody for the TN-XXL expression and an anti-GAPDH antibody as control. ( c ) Images of three newborn mice (HO, homozygous; HE, heterozygous; WT, wild-type) illuminated with bright field (monochrome), CFP (blue) and cpCitrine (yellow) fluorescence. ( d ) Bright field and fluorescence images of isolated organs from TN-XXL transgenic mice (right) compared with wild-type controls (left). ( e ) Overview of TN-XXL fluorescence (green) in frozen sections of several tissues co-stained with 4′,6-diamidino-2-phenylindole (DAPI; magenta) (Scale bars, 500 μm). Full size image Despite the ubiquitous promoter, high-resolution composite images of cryo-sectioned organs revealed differential TN-XXL expression and showed tissues, which lack expression but only showed 4′,6-diamidino-2-phenylindole (DAPI) counter-staining ( Fig. 1e ). Most notably lymph follicles in spleen, lymph nodes and thymus of transgenic mice were completely devoid of TN-XXL expression while connective tissues within these organs showed bright expression ( Fig. 1e ; Supplementary Fig. S2A ). Detailed analysis of lymphocytes from lymph nodes, thymus and bone marrow by flow cytometry revealed no TN-XXL-positive immune cells ( Supplementary Fig. S2B ). In comparison with kidney cells, total spleen cells showed highly reduced TN-XXL messenger RNA levels ( Supplementary Fig. S2C ), suggesting a silencing of transgene transcription specifically in the majority of hematopoietic cell types. Surprisingly, a significant percentage of platelets (about 30%) were found by flow cytometry to express TN-XXL at detectable levels (Claudia Nußbaum, Mark Sperandi, personal communication). Interestingly, several areas associated with neurogenesis of the adult brain, such as the dentate gyrus and the subventricular zones, appeared to show mostly DAPI staining but little or lack of TN-XXL expression ( Fig. 1e ). Indicator concentration and mobility inside cells To calculate the TN-XXL concentration in specific tissues, we generated a calibration standard curve using purified TN-XXL ( Fig. 2a ; Supplementary Fig. S3A , Supplementary Methods ) and compared its fluorescence intensity with acute sections from tissues of homozygous transgenic mice. Calculated TN-XXL concentrations were determined in hippocampal blood vessels (4.2 μM±0.7 (s.d. )), hippocampal neurons (2.3 μM±0.3 (s.d. )), kidney (3.2 μM±1.0 (s.d.)) and in liver (1.2 μM±0.2 (s.d.)) ( Fig. 2b ). The high s.d. in kidney is caused by the large variety of expression levels in different cell types that were not further identified. In muscle and heart tissue three subsets of expressing fibers (low, medium and high) were observed ( Fig. 2b ). In muscle tissue a concentration of TN-XXL from 2.4 to 5.7 μM was calculated. In heart tissue levels were in the same range. The generation of histograms of the analysed tissues helped to confirm the distribution into three subsets ( Supplementary Fig. S3B,C ). An important limitation of biosensors expressed inside cells might be aggregation or binding to components of the cytosol, thereby reducing the sensors' free mobility and diffusion. Indeed, in a transgenic mouse line stably expressing the calmodulin-based sensor YC 3.12 the sensor had lost calcium sensitivity and showed punctuate immobile fluorescence of a large fraction of the sensor population [17] . To test for free diffusion and mobility of TN-XXL fluorescence recovery after photo bleaching (FRAP) experiments were carried out in cultured murine kidney fibroblasts (MKF) prepared from homozygous transgenic mice ( Fig. 2c ). The recovery rate ( t ) of 0.2 s after the bleaching pulse taken at a relatively slow frame rate of 4 Hz was in line with rates obtained for GFP [29] and suggested free mobility and diffusion of TN-XXL ( Fig. 2d ). Furthermore, we tested whether TN-XXL expressed long-term via transgenic methods had properties comparable to TN-XXL acutely transfected into cells overnight. Therefore, cultured MKF isolated from transgenic mice were compared with wild-type MKF transfected overnight with an expression plasmid coding for TN-XXL. Baseline ratios had similar values for transfected wild-type and transgenic cells of ~1±0.1 (s.d) ( Fig. 2e , left). Agonist-induced responses in fibroblasts from transgenic mice and wild-type fibroblasts acutely expressing the indicator for 16 h were indistinguishable ( Fig. 2e , right). In addition, we investigated whether long-term expression of TN-XXL could cause changes in cell morphology. In a previous study a pathological aggregation of several GECIs to the nucleus was reported after long-term adeno-associated virus vector-mediated expression in cortical neurons [11] . Here, we looked at 13 days, 36 days, 2-month- and 6-month-old brains from TN-XXL transgenic mice and performed confocal images of frozen sections of the CA1 and CA3 region of the hippocampus ( Supplementary Fig. S4A ). We examined the cytosolic and nuclear fluorescence distribution by drawing a line through the soma of neurons ( Supplementary Fig. S4B ). Statistical analysis revealed no nuclear aggregation of TN-XXL in CA1 and CA3 neurons ( Supplementary Fig. S4C ). 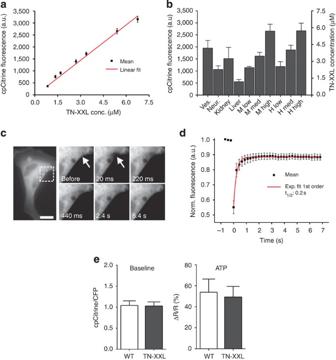Figure 2: TN-XXL concentration and functionality in cells of TN-XXL transgenic mice. (a,b) Concentration determination of TN-XXL. (a) Calibration curve using recombinant purified TN-XXL dilutions (mean±s.d,n=4). (b) Estimation of TN-XXL protein concentrations in cells of acute slices (400 μm) from brain (Ves., blood vessels; Neur, hippocampal neurons), kidney, liver, and for low, medium (med) and high expressing fibers of muscle (M) and heart (H). (c,d) FRAP experiments in cultured MKF of TN-XXL transgenic mice. (c) Fluorescence images of a kidney fibroblast. Blow-ups show the region marked with a white rectangle in the left picture. Arrows indicate the site of the bleached spot at indicated time points after bleaching (Scale bar, 15 μm). (d) Time course of fluorescence recovery after photobleaching (mean±s.e.m.,n=3). (e) Functionality of TN-XXL in cultured MKF (mean±s.e.m,n=3). Fibroblasts from TN-XXL transgenic mice and from wild-type mice acutely transfected overnight with TN-XXL were compared. (e, left) Ratio for basal calcium of transgenic (TN-XXL) and wild-type MKF (WT) expressing TN-XXL. (e, right) Comparison of average agonist evoked responses for application of ATP in fibroblasts. Figure 2: TN-XXL concentration and functionality in cells of TN-XXL transgenic mice. ( a , b ) Concentration determination of TN-XXL. ( a ) Calibration curve using recombinant purified TN-XXL dilutions (mean±s.d, n =4). ( b ) Estimation of TN-XXL protein concentrations in cells of acute slices (400 μm) from brain (Ves., blood vessels; Neur, hippocampal neurons), kidney, liver, and for low, medium (med) and high expressing fibers of muscle (M) and heart (H). ( c , d ) FRAP experiments in cultured MKF of TN-XXL transgenic mice. ( c ) Fluorescence images of a kidney fibroblast. Blow-ups show the region marked with a white rectangle in the left picture. Arrows indicate the site of the bleached spot at indicated time points after bleaching (Scale bar, 15 μm). ( d ) Time course of fluorescence recovery after photobleaching (mean±s.e.m., n =3). ( e ) Functionality of TN-XXL in cultured MKF (mean±s.e.m, n =3). Fibroblasts from TN-XXL transgenic mice and from wild-type mice acutely transfected overnight with TN-XXL were compared. ( e , left) Ratio for basal calcium of transgenic (TN-XXL) and wild-type MKF (WT) expressing TN-XXL. ( e , right) Comparison of average agonist evoked responses for application of ATP in fibroblasts. Full size image Calcium responses in dissociated primary cell types Transgenic mice stably expressing TN-XXL could be a useful source of primary cell types ready for various calcium imaging or drug screening applications. We therefore tested the functionality of TN-XXL in three primary cell types. We isolated and cultured smooth muscle cells (SMC) from bladder, fibroblasts from kidney and astrocytes from cortical tissue of homozygous transgenic mice ( Fig. 3a ). All cell types showed fluorescence for at least 8 weeks in culture (data not shown). SMC responded to application of carbachol (100 μM) with an average peak response of ~30% Δ R / R and ongoing calcium oscillations for several minutes ( Fig. 3b , top). Calcium responses with ratio changes of up to 60% Δ R / R were elicited in MKF after bath application of ATP (10 μM) ( Fig. 3b , bottom). When ATP (10 μM) was applied to cultured astrocytes oscillations were also detected. Older, denser astrocyte cultures showed a high rate of spontaneous oscillations. ATP increased the oscillation frequency over the time of application ( Fig. 3b , right). 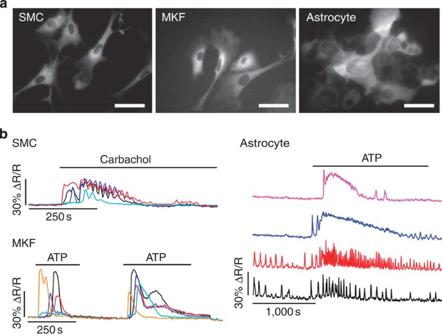Figure 3: Calcium responses in primary cell types of TN-XXL transgenic mice. (a) Fluorescence images of aortic SMC, MKF and astrocytes (Scale bars, 25 μm). (b) Agonist-induced calcium responses in SMC (Carbachol, 100 μM), MKF (ATP, 10 μM) and astrocytes (ATP, 10 μM) in younger (upper traces) or older (lower traces) cultures. Colours represent traces of individual cells. Figure 3: Calcium responses in primary cell types of TN-XXL transgenic mice. ( a ) Fluorescence images of aortic SMC, MKF and astrocytes (Scale bars, 25 μm). ( b ) Agonist-induced calcium responses in SMC (Carbachol, 100 μM), MKF (ATP, 10 μM) and astrocytes (ATP, 10 μM) in younger (upper traces) or older (lower traces) cultures. Colours represent traces of individual cells. Full size image Calcium imaging in tissue explants Organ explants offer ease of pharmaceutical manipulation for research and drug screening applications, retain tissue context and thus are a first approximation to in vivo work. Isolated branches of the mesenteric artery system are used in many pharmacological studies of the vascular system [30] , [31] , [32] . In mesenteric artery explants from TN-XXL transgenic mice, expression was predominantly found in endothelial cells, with SMC only occasionally showing detectable expression ( Fig. 4a ). Fluorescence was lining the blood vessel lumen where endothelial cells expressed. As expected their nuclei were devoid of fluorescence ( Fig. 4a ). Using confocal microscopy we performed calcium-imaging experiments in these endothelial cells of an artery explant. Bath application of acetylcholine (3 μM), a vasoconstrictor, elicited long lasting calcium transients in mesenteric endothelial cells with up to 80% Δ R / R ( Fig. 4b ). In total 37% of cells ( n =75) responded to acetylcholine in this preparation (data not shown). 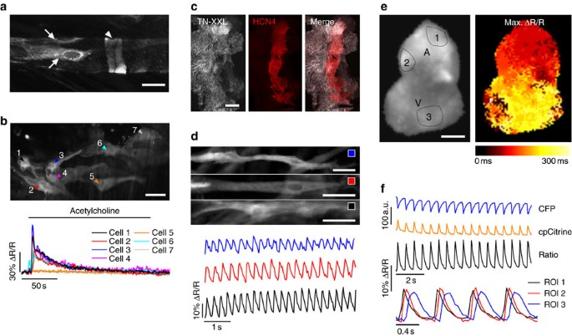Figure 4: Calcium imaging in tissue explants of TN-XXL mice. (a,b) Calcium imaging in mesenteric arteries. (a) Fluorescence image of a mesenteric blood vesselin vivoshowing TN-XXL expressed in endothelia (arrows) and SMC (arrowhead). (b)Ex vivocalcium imaging of seven endothelial cells in a mesenteric artery explant. The graph below shows the calcium responses upon application of 3 μM acetylcholine (Scale barsa,b, 25 μm). (c,d) Immunocytochemistry and calcium imaging of the SAN region of the mouse heart. (c) Immunocytochemistry of SAN explants. The left image illustrates cpCitrine fluorescence, the image in the middle highlights the staining with anti-HCN4 antibodies, a marker of the SAN (red). Right merged image shows co-localization (Scale bar, 500 μm). (d) Calcium imaging of cells in SAN explants. 30 Hz high-speed imaging of three cells (blue, red and black) from three different spontaneously beating SAN explants recorded at 30 °C (Scale bars, 25 μm). (e,f) Wide-field calcium imaging of whole embryonic hearts of TN-XXL transgenic mice. (e) Fluorescence image of a day 8.5 embryonic heart (left). Dotted circles refer to the regions of interest (ROIs) plotted in (f) (A, atria; V, ventricles). The phase plot in the right picture illustrates the progression of the calcium signal over one heartbeat cycle. The colour code indicates the time at which the maximum ΔR/Rwas observed at a given pixel (Scale bar, 150 μm). (f) Calcium transients of spontaneous beatings recorded from the heart shown in (e). Shown are intensities of CFP (blue) and cpCitrine (orange) emission channels (ROI 1) and the corresponding ratio (black). The lower graph shows a blow-up of four beating cycles for the indicated ROIs. Figure 4: Calcium imaging in tissue explants of TN-XXL mice. ( a , b ) Calcium imaging in mesenteric arteries. ( a ) Fluorescence image of a mesenteric blood vessel in vivo showing TN-XXL expressed in endothelia (arrows) and SMC (arrowhead). ( b ) Ex vivo calcium imaging of seven endothelial cells in a mesenteric artery explant. The graph below shows the calcium responses upon application of 3 μM acetylcholine (Scale bars a , b , 25 μm). ( c , d ) Immunocytochemistry and calcium imaging of the SAN region of the mouse heart. ( c ) Immunocytochemistry of SAN explants. The left image illustrates cpCitrine fluorescence, the image in the middle highlights the staining with anti-HCN4 antibodies, a marker of the SAN (red). Right merged image shows co-localization (Scale bar, 500 μm). ( d ) Calcium imaging of cells in SAN explants. 30 Hz high-speed imaging of three cells (blue, red and black) from three different spontaneously beating SAN explants recorded at 30 °C (Scale bars, 25 μm). ( e , f ) Wide-field calcium imaging of whole embryonic hearts of TN-XXL transgenic mice. ( e ) Fluorescence image of a day 8.5 embryonic heart (left). Dotted circles refer to the regions of interest (ROIs) plotted in ( f ) (A, atria; V, ventricles). The phase plot in the right picture illustrates the progression of the calcium signal over one heartbeat cycle. The colour code indicates the time at which the maximum Δ R / R was observed at a given pixel (Scale bar, 150 μm). ( f ) Calcium transients of spontaneous beatings recorded from the heart shown in ( e ). Shown are intensities of CFP (blue) and cpCitrine (orange) emission channels (ROI 1) and the corresponding ratio (black). The lower graph shows a blow-up of four beating cycles for the indicated ROIs. Full size image The sinoatrial node (SAN) is the pacemaker region of the mammalian heart [33] . We established a SAN preparation from the adult TN-XXL mouse heart and used it for confocal calcium imaging. To verify correct dissection of the SAN we performed immunostainings using antibodies against the hyperpolarization activated ion channel HCN4, a marker for pace-maker cells of the SAN [34] ( Fig. 4c ). Living SAN explants were analysed with single-cell resolution at an imaging frequency of 30 Hz. Cells were beating at frequencies of up to 4 Hz under these conditions and corresponding calcium signals could readily be recorded ( Fig. 4d ). Motion artifacts owing to the high beating frequencies were well cancelled out due to the ratiometric readout of TN-XXL. Wide field fluorescence CCD (charge-coupled device) camera imaging allows investigating large-scale organization of calcium signals in a living organ. To demonstrate usefulness of tissues prepared from TN-XXL mice for this purpose we dissected whole hearts from embryonic day 8.5 mice [35] and cultured them for up to 2 days. Calcium waves travelling through the organ over a distance of about 800 μm with every heartbeat could be readily recorded. The ratiometric nature of TN-XXL facilitated imaging in this moving organ preparation. The propagation of the calcium wave from the atria (A) to the ventricles (V) is illustrated by a phase plot of one beating cycle in Fig. 4e (right). The curve progression in regions of interests picked in the atrial and ventricular region ( Fig. 4e , left) demonstrated the temporal delay of the conduction of the calcium signal from the atria to the ventricles ( Fig. 4f , lower graph and Supplementary Fig. S5 ). Expression profiling of TN-XXL transgenic mice It has been debated whether expression of GECIs over long periods of time could induce phenotypes in host cells and organisms over time. This could potentially be due to enhanced calcium buffering or to some residual signalling that is inherent to the calcium-binding domain used to construct the sensor. To generate a validated mouse model we therefore decided to look into potential effects of global long-term TN-XXL expression on the mouse. Altered patterns of gene expression are a crucial hallmark of homeostatic responses of an organism. Indeed, many stress-inducing conditions or disease states can lead to changes in the regulation of large numbers of genes. Using transcriptional profiling we therefore analysed large-scale global mRNA expression levels in muscle, heart (the tissues with highest TN-XXL expression) and in hippocampus of TN-XXL transgenic mice to identify potential genes that could be regulated in response to TN-XXL expression. Transcript expression levels in transgenic mice were compared with those of non-transgenic littermates. We found a large number of genes with mild levels of regulation (<2-fold) that were not considered physiologically relevant ( Supplementary Fig. S6 and Supplementary Data ). In total, we found an upregulation of 102, 42 and 0 genes and a downregulation of 173, 33 and 0 genes for skeletal muscle, heart and hippocampus, respectively (>2-fold regulation) (see Supplementary Fig. S6 and Supplementary Data ). Ten genes with the highest levels of regulation in heart and skeletal muscle are summarized in Table 1 . In hippocampus no gene with significantly altered regulation above threshold was detected. Most notable is the significant 8-fold induction of transcripts coding for metallothionein-2 in muscle, and a smaller 2.7-fold induction was also observed in the heart ( Table 1 ). Metallothionein-2 is a zinc and copper-binding protein that has been suggested to have a role in protection against oxidative damage [36] , but its detailed cellular role is to date unknown. It might be speculated that this gene and possibly some of the other detected genes are induced to deal with reactive oxygen species generated during GFP chromophore formation [37] . Table 1 Genes regulated in TN-XXL mice. Full size table Telemetric electrocardiograms in TN-XXL transgenic mice To determine whether TN-XXL overexpression affected the electrical activity of the heart, we recorded in vivo telemetric long-term ECG in freely moving TN-XXL and wild-type mice ( Fig. 5a ). In long-term measurements over 24 h, TN-XXL mice revealed a regular sinus rhythm with no evidence for spontaneous arrhythmias. TN-XXL transgenic mice had indistinguishable minimum heart rates but showed lower mean heart rates and maximal heart rates compared with controls ( Fig. 5b ). Heart rate histograms showed that low heart rates were more frequent in TN-XXL transgenic mice than in wild-type mice ( Supplementary Fig. S7 ). In addition, beta-adrenergic stimulation achieved by intraperitoneal injection of isoprenaline did not lead to the same increase of the heart rate in TN-XXL transgenic mice compared with wild-type controls ( Fig. 5b ) indicating chronotropic incompetence of TN-XXL transgenic mice. 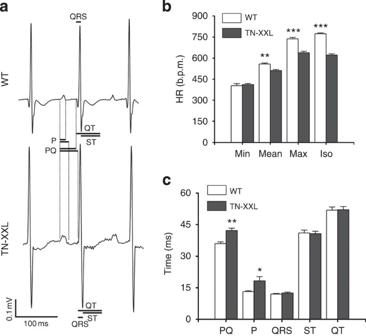Figure 5: Long-termin vivotelemetric ECG in adult TN-XXL transgenic mice. (a) Representative lead II ECG traces of TN-XXL and WT mice obtained by telemetric measurements at a resting heart rate of 500 b.p.m. Definitions of the ECG parameters (PQ, P, QRS, ST, QT) are indicated as specified in the methods section. Note the biphasic and prolonged p wave indicating atrial hypertrophy. (b) Heart rate analysis of transgenic (TN-XXL) and wild-type controls (WT). Minimum (min), mean and maximum (max) heart rates were calculated from the 24 h ECG. Iso=maximum heart rate after i.p. injection of isoprenaline (0.1 mg kg−1body weight). (c) ECG parameters at a heart rate of 500 b.p.m. Letters on theXaxis refer to the different phases in the ECG as indicated in panel A. Throughout, error bars represent SEM; *P<0.05; **P<0.01; ***P<0.001;n=6 mice per group. Significance was tested by analysis of variance (ANOVA) followed by Dunett test. Figure 5: Long-term in vivo telemetric ECG in adult TN-XXL transgenic mice. ( a ) Representative lead II ECG traces of TN-XXL and WT mice obtained by telemetric measurements at a resting heart rate of 500 b.p.m. Definitions of the ECG parameters (PQ, P, QRS, ST, QT) are indicated as specified in the methods section. Note the biphasic and prolonged p wave indicating atrial hypertrophy. ( b ) Heart rate analysis of transgenic (TN-XXL) and wild-type controls (WT). Minimum (min), mean and maximum (max) heart rates were calculated from the 24 h ECG. Iso=maximum heart rate after i.p. injection of isoprenaline (0.1 mg kg −1 body weight). ( c ) ECG parameters at a heart rate of 500 b.p.m. Letters on the X axis refer to the different phases in the ECG as indicated in panel A. Throughout, error bars represent SEM; * P <0.05; ** P <0.01; *** P <0.001; n =6 mice per group. Significance was tested by analysis of variance (ANOVA) followed by Dunett test. Full size image To investigate the dynamics of heart rate oscillations we performed a heart rate variability analysis ( Supplementary Figs S8 and S9 , Supplementary Methods ). Electrocardiograms (ECG) and tachograms of wild-type mice showed a broad variation of the RR interval ( Supplementary Fig. S8A,B ). These beat-to-beat fluctuations in heart rate are generated by the opposing effects of sympathetic and parasympathetic input. A similar range of fluctuations in the heart rate has been known in the literature for wild-type mice. In contrast to wild-type mice, in TN-XXL these broad range fluctuations were not present. In TN-XXL the RR interval hardly changed over time ( Supplementary Fig. S8A,B ). To directly compare heart rate-dependent ECG parameters, we analysed the ECG during episodes of a defined heart rate of 500 beats per minute. We found prolonged PQ intervals in transgenic mice ( Fig. 5a,c ), indicating a first degree AV block. In addition, P waves in TN-XXL transgenic mice ( Fig. 5a,c ) were prolonged and had a biphasic shape suggesting atrial hypertrophy. Consistent with this right and left atria weights as well as atrial size and cell diameters were slightly increased in TN-XXL mice ( Supplementary Table S1 , Supplementary Fig. S10 ). It has been previously shown that in transgenic mice that overexpress GFP [38] , the Ca 2+ binding protein calmodulin [39] or G-CaMP2 (ref. 18 ) cardiac hypertrophy is induced. Interestingly, in the latter it has been shown that cardiac hypertrophy could be avoided when using inducible transgene expression and limiting experiments to a short time window after on-set of expression. No difference was detected in QRS, ST and QT intervals. There was no difference between the QT c of wild-type (47.37±1.3 ms ( n =6)) and TN-XXL mice (47.44±1.4 ms n =6). The amplitudes of p-wave, r-wave and s-wave were normal. Together these data notify that ventricular conduction and repolarization were unaltered in TN-XXL transgenic mice ( Fig. 5c ). Overall, a potential signature of indicator expression is a chronotropic incompetence, atrial hypertrophy and slower atrioventricular conduction in TN-XXL transgenic mice. Behavioural testing of TN-XXL transgenic mice Behaviour is the result of a multitude of physiological and cognitive processes that have to be coordinated and fine-tuned within the organism. Thus, behavioural performance appeared to be a suitable read-out to test whether global TN-XXL expression leaves a detectable behavioural phenotype. We performed a battery of different behavioural tasks for motor behaviour, emotionality, learning and memory, and depression-related behaviour and compared homozygous TN-XXL transgenic mice with wild-type littermates. Tests monitoring exploratory, motor behaviour and skilled movements were performed, taking into consideration the pronounced expression of TN-XXL in muscle, motoneurons and all cortical cerebral areas. The exploratory hole board test revealed no differences between TN-XXL transgenic mice and wild-type mice in any of the explored parameters ( Fig. 6a ). In addition, the rotarod test, a task for motor coordination, skilled movements and motor learning, did not reveal any significant differences ( Fig. 6b ). In contrast, if tested in an exploration-based paradigm of innate anxiety, TN-XXL transgenic mice showed an increased exploration of the aversive open arms of the elevated plus-maze ( t =2.56; P <0.05), which cannot be explained by changes in locomotor activity ( Fig. 6c ). In addition, they spent more time in social investigation ( t =3.80; P <0.01) than wild-type littermate controls ( Fig. 6d ). Together, these data indicate a decrease in anxiety-like behaviour in TN-XXL transgenic mice, which, however, was not evident in the light-dark test, if the number of entries into (wild-type=35.5±3.6%; TN-XXL=41.8±1.5%, P >0.05) and the time spent in the light compartment (wild-type=21.3±2.8%; TN-XXL=27.6±4.9%, P >0.05) were considered (data not shown). There was an increase in arousal, as revealed in the acoustic startle paradigm ( Fig. 6e ). Acquisition of auditory cues and contextual fear memory, in contrast were unaffected by the transgene ( Fig. 6f ; factor genotype: P >0.05). Nevertheless, TN-XXL transgenic mice showed an accelerated decline of conditioned fear upon prolonged re-exposure to the tone ( Fig. 6f ; genotype × interval: F 8,264 =3.67, P <0.001; two-way analysis of variance). Finally, TN-XXL mice were less immobile in the tails suspension test ( Fig. 6g ; t =2.18; P <0.05), which measures depression-like behaviour. All in all, TN-XXL transgenic mice showed normal motor behaviour and were undisturbed in motor learning and hippocampus- and amygdala-dependent classical fear conditioning. However, they were less anxious and more readily acquired active coping strategies in stressful situations. 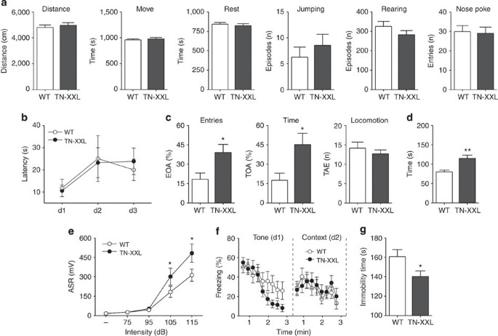Figure 6: Behavioural characterization of TN-XXL transgenic mice and wild-type controls (WT). (a) Hole board test. Distance covered, distance in time, resting, jumping, rearing behaviour and the number of nose pokes were analysed during a 30-min monitoring period. (b) Rotarod. Mice were placed on accelerating drums. The time at which an animal fell from the drum was measured. The increased latency from day 1 (d1) to day 2 (d2) and day 3 (d3) indicates motor learning behaviour. (c) Elevated plus maze (EPM). Time spent in open arm (TOA), entries in open arm (EOA) and locomotion as motility control was analysed. (d) Social interaction test (SI). Pairs of unfamiliar mice (n=7 pairs each) were placed into a new environment. The time of active contacts (sniffing, licking, close following, grooming) was recorded. (e) Acoustic startle response (ASR). To test for hyperarousal, startle stimuli consisted of white noise bursts of 75, 90, 105 and 115 dB were applied. (f) Fear conditioning test. Mice were placed into a shock chamber and a tone was presented followed by an electric foot shock. After conditioning, mice were exposed either to the tone in neutral environment (d1) or to the shock chamber without applying an electric shock (d2). Freezing behaviour served as a measure of fear memory. (g) Tail-suspension test. Mice were suspended by the tail from a metal rod and the immobility times during the last 4 min of the 6 min trial period was recorded. Data in all graphs are shown as mean±s.e.m. (sample sizes were 12–15 animals for each test). Figure 6: Behavioural characterization of TN-XXL transgenic mice and wild-type controls (WT). ( a ) Hole board test. Distance covered, distance in time, resting, jumping, rearing behaviour and the number of nose pokes were analysed during a 30-min monitoring period. ( b ) Rotarod. Mice were placed on accelerating drums. The time at which an animal fell from the drum was measured. The increased latency from day 1 (d1) to day 2 (d2) and day 3 (d3) indicates motor learning behaviour. ( c ) Elevated plus maze (EPM). Time spent in open arm (TOA), entries in open arm (EOA) and locomotion as motility control was analysed. ( d ) Social interaction test (SI). Pairs of unfamiliar mice ( n =7 pairs each) were placed into a new environment. The time of active contacts (sniffing, licking, close following, grooming) was recorded. ( e ) Acoustic startle response (ASR). To test for hyperarousal, startle stimuli consisted of white noise bursts of 75, 90, 105 and 115 dB were applied. ( f ) Fear conditioning test. Mice were placed into a shock chamber and a tone was presented followed by an electric foot shock. After conditioning, mice were exposed either to the tone in neutral environment (d1) or to the shock chamber without applying an electric shock (d2). Freezing behaviour served as a measure of fear memory. ( g ) Tail-suspension test. Mice were suspended by the tail from a metal rod and the immobility times during the last 4 min of the 6 min trial period was recorded. Data in all graphs are shown as mean±s.e.m. (sample sizes were 12–15 animals for each test). Full size image Here, we describe the generation and validation of a transgenic mouse model expressing the calcium biosensor TN-XXL using the ubiquitous CAG promoter. We find widespread expression of the sensor in a large number of cell types and organs, with noticeable exceptions being cell lineages of the hematopoietic system other than thrombopoiesis. In all expressing cell types tested the sensor was functional and localized to the cytosol. Importantly, there was no pathological nuclear translocation of the sensor in hippocampal CA1 neurons of mice from age postnatal day 13 to 6-month-old animals. By contrast, studies on long-term expression of several GECIs by adeno-associated virus-mediated gene transfer recently reported progressing cytomorbidity and concomitant restricted localization of the sensor to the cell nucleus [11] . Thus, transgenic expression of calcium biosensors is likely to be more suitable for long-term expression of indicators. A particular focus of this study was on biocompatibility of the sensor, an aspect that deserves more attention in studies to characterize GECI function in vivo . We used microarray expression profiling, anatomical analysis, behavioural testing and recording of basic physiological parameters to assess potential consequences of biosensor expression on the host organism. The vast majority of parameters tested did not differ between TN-XXL transgenic mice and non-transgenic littermates. We did, however, identify potential signatures of indicator expression that were mild and may also relate to positional effects upon integration of the transgene into the genome, but are worth to be taken into account. On the behavioural level TN-XXL transgenic mice showed a specific altered behaviour in a limited number of test batteries related to neurological disorders, such as fear conditioning or the elevated plus maze. Interestingly, recent evidence hints at a role of calcium-mediated mechanisms in modulating plasticity along the thalamus-amygdala pathway [40] that underlies some of these behaviours. TN-XXL expression had detectable effects on cardiac physiology, in particular a chronotropic incompetence, slight atrial hypertrophy and slower atrioventricular conduction in TN-XXL transgenic mice. TN-XXL transgenic mice had normal minimal heart rates. TN-XXL expression, however, caused a reduced maximal heart rate under maximal adreneric stimulation, thus reducing the overall dynamic range of heart rate regulation. It is possible that overexpression of TN-XXL buffers Ca 2+ in SAN pacemaker cells, which is required to increase the slope of the pacemaker potential [41] and is utilized to support the physiological increase in heart rate. In line with this hypothesis it has been shown that chelating SAN Ca 2+ by EGTA [41] , BAPTA [41] or the Ca 2+ indicator Indo-1 (refs 42 , 43 ) significantly reduces the slope of diastolic depolarization and beating rate of sinoatrial pacemaker cells. Using expression profiling we could detect a number of transcripts regulated predominantly in heart and skeletal muscle of TN-XXL transgenic mice but only very few showed a level of regulation of a factor of two or higher and thus the majority of these changes were considered physiologically irrelevant. Remarkably this regulation occurred in skeletal and cardiac muscle, but not in brain. This finding suggests that skeletal muscle TnC as calcium sensing moiety within the indicator may be bio-orthogonal in brain but may lose some of this advantage in muscle tissue where it is derived from. The transcript with the highest level of regulation (8-fold induction in skeletal muscle) was the gene coding for metallothionein-2. This protein was reported to bind zinc and copper and is considered to have a role in protection against oxidative damage [36] . Further details on the physiological role of metallothionein-2 are not known. Perhaps it may be induced to deal with reactive oxygen species generated during GFP chromophore formation [37] . A recent study reported that high level expression of yellow fluorescent protein (YFP) in a thy1 -YFP reporter mouse line induced a significant up regulation of more than 40 genes involved in cell stress activation, apoptosis and inflammation [44] . In summary, long-term expression of TN-XXL in transgenic mice thus seems to be well tolerated, results in fully functional sensor even after months of transgenic expression and in all cell types analysed so far, and induces only a mild and subtle signature in some specific instances. The data also suggest that it may be worthwhile to further optimize biocompatibility of sensor design. Further improvements in indicator design may arise from minimizing the calcium binding domain and reducing the number of EF-hands necessary to generate a large FRET change. This reduces calcium buffering caused by the indicator and potential residual biological activity of the sensing domain. Other improvements may arise from incorporating brighter fluorescent protein variants, such as mCerulean3 [45] or mTurquoise [46] , to allow lower expression levels while maintaining the same signal-to-noise levels. The data on biocompatibility give guidance for further developments and use of calcium biosensors, and the mice generated provide a valuable validated resource of primary cells and tissues for in vitro and in vivo calcium imaging applications. It is plausible that the mouse model generated here might be useful in combination with many mouse disease models available to date. Chronic long-term functional imaging studies with GECIs with established biocompatibilities such as TN-XXL and its updates thus could offer exciting new possibilities to follow physiologies of cells and tissues as they differentiate, adapt to stimuli and degenerate due to ageing and disease. Mice To facilitate placing TN-XXL under control of the β-actin promoter we integrated a multiple cloning site (MCS) into the pCAG expression vector [27] . pCAG was linearized by restriction digestion with Eco RI, dephosphorylated and a double-stranded DNA oligonucleotide containing various restriction sites was integrated to generate pCAG-MCS. The WPRE [28] was placed downstream of TN-XXL. To this end WPRE was amplified by PCR, cut by Eco RI and Xho I and ligated into pcDNA3-TN-XXL cut by the same enzymes, giving rise to pcDNA3-TN-XXL-WPRE. From this vector TN-XXL-WPRE was released by digestion with Not I and Xho I and ligated into pCAG-MCS opened by the same enzymes, eventually yielding pCAG-TN-XXL-WPRE. For generation of TN-XXL transgenic mice, pCAG-TN-XXL-WPRE was linearized with Ssp I and Hind III, purified and microinjected into the pronuclei of fertilized C57BL/6N oocytes. All animal procedures used in this report were in accordance with guidelines of the committee on animals of the Max Planck Institute of Neurobiology and with the license of the Regierung von Oberbayern (Munich, Germany). Imaging of primary cultured cells Cells were grown on poly-l-lysine coated glass-bottom dishes (MatTek Corp., MA, USA) and imaged with a Zeiss Axiovert 35 M inverted microscope equipped with a CCD camera (Photometrics CoolSnap, Roper Scientific, Germany). The imaging setup was controlled by Metafluor version 4.6 software (Universal Imaging, Sunnyvale, CA, USA). For ratiometric imaging, a 440/20-excitation filter, a 455 dichroic long-pass mirror and two emission filters (485/35 for enhanced cyan fluorescent protein (eCFP), 535/25 for cpCitrine) operated in a filter wheel (Sutter Instruments, Novata, CA, USA) were used. All filters were purchased from Chroma Technology Corp (Bellow Falls, VT, USA). Confocal calcium imaging of SAN cells After dissection SAN explants were pinned on a custom built temperature controlled stage and equilibrated to 30 °C. Single- cell calcium imaging was performed on a TPS 5 SPII laser scanning confocal microscope (Leica Microsystems, Wetzlar, Germany) using 458 nm argon ion laser excitation at 20% output power and acousto-optic tunable filter levels of 30% with a low magnifying X20/0.5 NA water immersion objective (Leica Microsystems) at a scan speed of 1,400 Hz, which resulted in a frame rate of 30 Hz. Fluorescence emission was recorded with two photomultiplier tube (PMTs). The bandwidth of the CFP and cpCitrine emission channel was set to 465–505 nm at a PMT level of 750 V and 525–600 nm at a PMT level of 700 V, respectively. Concentration determination of TN-XXL expressing tissue TN-XXL was purified from E.coli . BL21 as described previously [22] . For higher purity high-performance liquid chromatography (ÄKTA Sweden) was applied with a Superdex 200 16/60 (GE Healthcare Europe, Germany) column and protein was concentrated with Amicon Ultra-15 (Millipore, MA, USA) to a concentration of 10 mg ml −1 (135 μM). This stock solution was diluted to 1:20, 1:25, 1:40, 1:50, 1:80, 1:100 and 1:160 for experiments. Organs (hippocampus, cortex, kidney, heart, hind limb muscle) of 4–8-month-old transgenic mice were cut into 400 μm thin section with a McIlwain tissue chopper (Mickle Laboratory Engineering Comp., Gomshall, England) and transferred to HBSS containing dishes until usage. The experiments were performed with a TCS SP5 II laser scanning confocal microscope (Leica Microsystems, Germany). Laser light of 514 nm at 17% output power and acousto-optic tunable filters of 15% were used for direct cpCitrine excitation of TN-XXL at a pinhole size of 80 μm. Images were recorded with a water immersion objective of ×20/0.5 NA at a scan speed of 400 Hz with a resolution of 1024×1024 pixels. The emission bandwidth was set to 525–600 nm with a PMT power of 650 V. These settings were used for all experiments. Microarrays For microarray analyses samples from hippocampus, heart and skeletal muscle from hind limb were used from three homozygous and three wild-type littermates. The tissue was dissected and shock-frozen in liquid nitrogen. RNA extraction and further analyses were performed by MFT Services (University of Tübingen, Germany). Briefly, RNA was isolated and 100 ng RNA per sample was amplified and marked with the GeneChip WT Terminal Labeling and Controls Kit (Ambion, Austin, TX, USA). Amplified and marked the RNA was hybridized on a MoGene 1.1 ST Gene Chip (Affymetrix Inc., Santa Clara, CA, USA), scanned with the GeneChip Scanner 3000 and analysed with the GeneChip Command Console Software AGCC 3.0 (Affymetrix Inc.). Fluorescence recovery after photo bleaching FRAP experiments were done with cultured transgenic murine kidney fibroblast (MKF) on a DeltaVision RT inverted microscope (Applied Precision, WA, USA) equipped with a quantifiable laser module at 488 nm and a CCD camera (CoolsnapHQ, Roper Scientific) for image capturing. Three images were taken before applying a photo bleaching laser pulse of 80 ms with a laser intensity of 50% at a defined bleaching area of about 25 μm 2 . After the pulse images were taken at a rate of 220 ms over a period of 8 s. Fluorescence intensity recovery was quantified and images were processed using ImageJ software. Behavioural experiments Male homozygous transgenic and control wild-type littermates ( n =12–15 per group) were used. Animals were single housed with food and water ad libitum under an inverse 12 h light/dark cycle. All behavioural experiments were performed during the activity phase of the mice between 0930 and 1700 hours and analysed blindly to the genotype of the animals. Data were analysed using unpaired t -test or two-factor analysis of variance for repeated measures and the post-hoc Newman–Keuls test for multiple comparisons. A P level of 0.05 or less was considered as indicative of a significant difference. For details on individual tests performed see Supplementary Information . Telemetric ECG recordings in mice Mice were housed in single cages in a 12 h dark/light cycle environment with free access to food and water. At the date of the surgery, the mice were at least 6 weeks old. Male TN-XXL transgenic mice and wild-type mice were anesthetized by intraperitoneal injection of ketamine and xylazine. An abdominal incision was made and radiotelemetric ECG transmitters (TA10ETA-F20, Data Sciences International, St Paul, MN, USA) were implanted into the peritoneal cavity. The ECG electrodes were place in a lead II configuration by suturing them s.c. onto the upper right chest muscle and the upper left abdominal wall muscle. Before measurements began, the mice were allowed to recover for 2 weeks. The analogue telemetric signals were digitized at 1 kHz and recorded by Dataquest A.R.T. 4.1 data acquisition software (Data Sciences International). For the 24 h ECG, data were sampled for 60 s every 30 min, for the drug injections, data were sampled continuously. Isoprenaline hydrochloride was dissolved in sterile 0.9% sodium chloride solution and injected intraperitoneal (0.1 mg kg −1 body weight). Data were analysed offline using Dataquest A.R.T. 4.0 data analysis software and Ponemah 4.8 ECG software (both by Data Sciences International). ECG parameters were measured semi-automatically and subsequently confirmed by a scientist. Both the drug injections and the ECG analysis were performed in a double-blinded fashion. The definitions of the ECG intervals are as follows: PQ: beginning of P to peak of Q; P: P-wave duration; QRS: peak of Q to peak of S; QT: peak of Q to end of T; ST: peak of S to end of T. In addition, the QT c interval was calculated to correct for heart rate according to Bazetta's formula (QTc=QT/((RR/100) 1/2 ) established for mice with QT interval and RR expressed in ms [47] . For details on analysis of heart rate variability and further additional methods consult Supplementary Information . Acccession codes: Microarray data have been deposited in Gene Expression Omnibus under accession code GSE39632 . How to cite this article: Direnberger, S. et al . Biocompatibility of a genetically encoded calcium indicator in a transgenic mouse model. Nat. Commun. 3:1031 doi: 10.1038/ncomms2035 (2012).